MEK inhibition reduced vascular tumor growth and coagulopathy in a mouse model with hyperactive GNAQ Activating non-inherited mutations in the guanine nucleotide-binding protein G(q) subunit alpha (GNAQ) gene family have been identified in childhood vascular tumors. Patients experience extensive disfigurement, chronic pain and severe complications including a potentially lethal coagulopathy termed Kasabach-Merritt phenomenon. Animal models for this class of vascular tumors do not exist. This has severely hindered the discovery of the molecular consequences of GNAQ mutations in the vasculature and, in turn, the preclinical development of effective targeted therapies. Here we report a mouse model expressing hyperactive mutant GNAQ in endothelial cells. Mutant mice develop vascular and coagulopathy phenotypes similar to those seen in patients. Mechanistically, by transcriptomic analysis we demonstrate increased mitogen activated protein kinase signaling in the mutant endothelial cells. Targeting of this pathway with Trametinib suppresses the tumor growth by reducing vascular cell proliferation and permeability. Trametinib also prevents the development of coagulopathy and improves mouse survival. Vascular anomalies are defects caused by the abnormal development and/or growth of the vasculature. Hyperactive postzygotic (noninherited) somatic mutations in the GNAQ gene (encoding the guanine nucleotide-binding protein G(q) subunit alpha or Gαq), or equivalent mutations in paralogous genes such as GNA11 and GNA14 , have been identified in a subset of vascular anomalies included in the classification proposed by the International Society for the Study of Vascular Anomalies (ISSVA) [1] , [2] . These include capillary malformation (CM)/Sturge-Weber syndrome (SWS), and a subset of vascular tumors, including congenital hemangioma (CH), tufted angioma (TA), kaposiform hemangioendothelioma (KHE) and pyogenic granuloma (PG) (also known as lobular capillary hemangioma) [1] , [2] , [3] , [4] . With the exclusion of CM and SWS, which are mostly associated with GNAQ mutations affecting arginine 183 (p.R183), vascular tumors are linked to GNAQ/11/14 mutation at glutamine 209 (p.Q209) (or equivalent p.Q205 in GNA14 ). Congenital hemangiomas affect newborns and can persist throughout life ( e.g . non-involuting congenital hemangioma or NICH). The other types of GNAQ/11/14 p.Q209-related vascular anomalies make their appearance during childhood and subsequently undergo proliferative expansion in these patients. Despite different ages of onset and life cycle, these vascular lesions are characterized by overlapping histopathological features. These include abnormal, structurally irregular lobules of proliferative and tightly packed endothelial cells (EC), and mildly enlarged capillaries and/or venules. The complications of this class of vascular anomalies are infection, infiltration to adjacent tissues such as muscle and bone, and cardiac overload leading to high-output heart failure. In addition, patients with TA or KHE can develop severe consumptive coagulopathy and thrombocytopenia (Kasabach-Merritt phenomenon or KMP) that is potentially lethal. KMP was first described in 1940 [5] in an infant affected by a rapidly enlarging vascular lesion associated with thrombocytopenia and hypofibrinogenemia, but the cellular and molecular events leading to KMP are still unknown. Current treatments for this subset of vascular anomalies include surgery, steroids, and vincristine [6] , while recent clinical trials have investigated the use of Sirolimus [7] , [8] . While surgery is the most effective intervention, often it is not indicated because of the increased risk of bleeding in these patients. Furthermore, due to the proliferative nature of these vascular tumors, surgery may not be curative. Gαq proteins (Gαq, Gα11, and Gα14) are members of the q class of G proteins that share about 90% sequence homology, and they mediate signals from G-protein-coupled receptors (GPCR) to phospholipase C-beta (PLC-β) [9] . They are normally expressed in different cell types, including vascular, blood and neuronal cells. Activated forms of Gα q and Gα 11 are frequent oncogenic drivers in uveal melanoma, an aggressive cancer of the adult eye, and they are also found in other melanocytic neoplasms [10] . As in vascular anomalies, these Gα subunits in uveal melanoma harbor a single amino acid substitution at Q209 or R183, which abrogates their intrinsic guanosine triphosphatase (GTPase) activity which normally serves to inactivate the protein. Therefore, gain-of-function, constitutively active mutants are thought to exist predominantly in the active, GTP-bound state. Studies in uveal melanoma have shown that this leads to hyperactivation of downstream effector molecules such as protein kinase C (PKC) and the mitogen-activated protein kinase (MAPK) cascade, which can lead to increased cellular proliferation [11] . To date, the EC-specific molecular and signaling consequences of hyperactive GNAQ are not well-defined, except for a handful of in vitro studies suggesting increased MAPK/ERK activity [2] , [4] , [12] . Furthermore, despite these genetic and mechanistic findings, genetic murine models for GNAQ -related vascular anomalies have not yet been reported. Here, we set out to create a murine model to study the etiology and pathogenesis of gain-of-function GNAQ -related vascular anomalies. We investigated the vascular, hematological, and transcriptomic consequences of endothelial expression of GNAQ p.Q209L. We further assessed a link between vascular morphogenesis defects, proliferation, permeability, and increased MAPK/ERK activation, in the mouse model and in patient-derived tissue. Finally, to establish the importance of the MAPK/ERK signaling in vascular pathology, we performed proof-of-concept preclinical experiments with a MEK/ERK inhibitor to assess its efficacy in extending mouse survival and preventing vascular lesion formation, growth, and coagulopathy. Endothelial-specific GNAQ Q209L expression during early postnatal development results in the formation of vascular abnormalities and vascular tufts To study the effects of hyperactive mutant GNAQ Q209L expression, we took advantage of a system that conditionally expresses human GNAQ p.Q209L in mice, the Rosa26-floxed stop-GNAQ Q209L line [13] . We first examined the effects of constitutive GNAQ Q209L expression by crossing Rosa26-floxed stop-GNAQ Q209L mice to the ubiquitously expressed CMV-Cre transgenic mouse [14] . Embryonic lethality was observed for the CMV-Cre; Rosa26-floxed stop-GNAQ Q209L genotype before embryonic day (E)8.5 (Supplementary Fig. 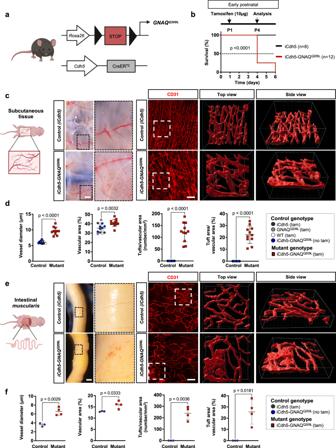Fig. 1: Early-onset vascular abnormalities and vascular tufts inGNAQQ209Lexpressing mice. aSchematic describing breeding scheme for generating models ofGNAQ-related vascular anomalies. TheRosa26-floxed stop-GNAQQ209Lmouse was crossed withCdh5-iCreERT2to generate EC specificGNAQQ209Lexpression (mutant mice are thereafter callediCdh5-GNAQQ209L).bSchematic describing Tamoxifen (tam) regimen for postnatal (P1) induction before experimental analysis of vasculature in the subcutaneous and intestinal tissue at P4. Kaplan-Meier curve comparing the survival percentage ofiCdh5-GNAQQ209L(n= 12, red) toiCdh5(n= 8, black) pups. Gehan–Breslow–Wilcoxon test (p< 0.0001).cLeft panel: Representative low- and high-power photographs of subcutaneous tissue from tamoxifen-treatediCdh5-GNAQQ209Land control pup (iCdh5). Scale bar: 2 mm. Right panel: Representative confocal z-stack images (max. intensity projection) of whole-mount staining for CD31 (red). The boxed regions (white dashed lines) are enlarged, and 3D reconstructed. Scale bar: 100μm.dQuantification of vessel diameter, vascular area as percentage of total area, tuft number as well as tuft area normalized to vascular area.iCdh5-GNAQQ209L(n= 11) and controls (n= 14), mean±SD, unpaired two-tailed Welch’s t-test. Mouse genotypes are indicated.eLeft panel: Representative low- and high-power photographs of intestinal tissue from tamoxifen-treatediCdh5-GNAQQ209Land control pup (iCdh5). Scale bar: 2 mm. Right panel: Representative confocal z-stack images (max. intensity projection) of whole-mount intestinalmuscularisstained for CD31 (red). The boxed regions (white dashed lines) are enlarged, and 3D reconstructed. Scale bar: 100μm.fQuantification of vessel diameter, vascular area as percentage of total area, tuft number, as well as tuft area normalized to vascular area.iCdh5-GNAQQ209L(n= 4) and controls (n= 3), mean±SD, unpaired two-tailed Welch’s t-test. Mouse genotypes are indicated. Source data for (b,d,f) are provided as a Source Data file. Schematic in (a,c,e) created with Biorender.com. 1 , Supplementary Table 1 ). Next, to test our hypothesis that endothelial GNAQ hyperactivation is sufficient to cause vascular anomalies, the Rosa26-floxed stop-GNAQ Q209L mouse line was crossed with the vascular EC specific and tamoxifen-inducible Cdh5-iCreER T2 [15] (or Pdgfb-iCreER T2 [16] , see Supplementary Figs. 4 , 5 , 7 ) to generate conditional GNAQ Q209L expression in EC (hereafter called iCdh5-GNAQ Q209L ). This system allows variable initiation of GNAQ Q209L expression, which occurs when Cre expression is induced upon the first injection of tamoxifen. To investigate the early postnatal vascular phenotypes caused by GNAQ Q209L in mice, we injected pups with tamoxifen at postnatal day 1 (P1) (Fig. 1a, b ). Fig. 1: Early-onset vascular abnormalities and vascular tufts in GNAQ Q209L expressing mice. a Schematic describing breeding scheme for generating models of GNAQ -related vascular anomalies. The Rosa26-floxed stop-GNAQ Q209L mouse was crossed with Cdh5-iCreER T2 to generate EC specific GNAQ Q209L expression (mutant mice are thereafter called iCdh5-GNAQ Q209L ). b Schematic describing Tamoxifen (tam) regimen for postnatal (P1) induction before experimental analysis of vasculature in the subcutaneous and intestinal tissue at P4. Kaplan-Meier curve comparing the survival percentage of iCdh5-GNAQ Q209L ( n = 12, red) to iCdh5 ( n = 8, black) pups. Gehan–Breslow–Wilcoxon test ( p < 0.0001). c Left panel: Representative low- and high-power photographs of subcutaneous tissue from tamoxifen-treated iCdh5-GNAQ Q209L and control pup ( iCdh5 ). Scale bar: 2 mm. Right panel: Representative confocal z-stack images (max. intensity projection) of whole-mount staining for CD31 (red). The boxed regions (white dashed lines) are enlarged, and 3D reconstructed. Scale bar: 100μm. d Quantification of vessel diameter, vascular area as percentage of total area, tuft number as well as tuft area normalized to vascular area. iCdh5-GNAQ Q209L ( n = 11) and controls ( n = 14), mean±SD, unpaired two-tailed Welch’s t-test. Mouse genotypes are indicated. e Left panel: Representative low- and high-power photographs of intestinal tissue from tamoxifen-treated iCdh5-GNAQ Q209L and control pup ( iCdh5 ). Scale bar: 2 mm. Right panel: Representative confocal z-stack images (max. intensity projection) of whole-mount intestinal muscularis stained for CD31 (red). The boxed regions (white dashed lines) are enlarged, and 3D reconstructed. Scale bar: 100μm. f Quantification of vessel diameter, vascular area as percentage of total area, tuft number, as well as tuft area normalized to vascular area. iCdh5-GNAQ Q209L ( n = 4) and controls ( n = 3), mean±SD, unpaired two-tailed Welch’s t-test. Mouse genotypes are indicated. Source data for ( b,d,f ) are provided as a Source Data file. Schematic in ( a,c,e ) created with Biorender.com. Full size image Human vascular anomalies caused by constitutively active GNAQ mutations are often localized to the skin or subcutaneous tissues [17] , [18] , [19] , [20] . Thereby, we harvested the subcutaneous tissue from the murine abdomen at P4, when 50% of mutant mouse lethality was detected (Fig. 1b ). Macroscopically, we detected vascular abnormalities in the mutant iCdh5-GNAQ Q209L mice (Fig. 1c ). The whole-mount subcutaneous tissue of iCdh5-GNAQ Q209L pups revealed abnormal and dilated CD31 + blood vessels (Fig. 1c and Supplementary Movies 1 , 2 ). Vessel diameter and vascular area were increased in iCdh5-GNAQ Q209L tissue compared to tamoxifen-injected littermates and mutant mice that did not receive tamoxifen (Fig. 1d ). In mutant mice, blood vessels were disorganized and formed lobules of abnormal, structurally irregular, and tightly packed vascular lesions, hereafter referred to as “vascular tufts”. For the analysis, we defined a vascular tuft as occupying an area ≥200 μm 2 . Tuft number and area were significantly increased (both at p < 0.0001) in the iCdh5-GNAQ Q209L tissues and were not detected in control tamoxifen-treated littermate tissue and in mutant mice that did not receive tamoxifen. Some of the GNAQ -related vascular tumors such as pyogenic granuloma and kaposiform hemangioendothelioma are often located in the gastrointestinal tract [21] , [22] , [23] . Macroscopically we detected vascular lesions in the intestine (Fig. 1e ). Therefore, we immunostained the murine intestinal muscularis for CD31. Whole-mount imaging analysis revealed the presence of vascular tufts in the intestinal muscularis of mutant mice (Fig. 1e ). Vessel diameter, vascular area, tuft number and tuft area were significantly ( p = 0.0029, p = 0.0333, p = 0.0036, and p = 0.0181 respectively) increased in iCdh5-GNAQ Q209L mice when compared to the intestinal muscularis of control mice (Fig. 1f ). To test the efficiency and specificity of the Cdh5-iCreER T2 driver, we crossed this mouse line with the Rosa26 tdTomato lineage reporter (hereafter called iCdh5-tdTomato ). Tamoxifen-induced activation of Cdh5-iCreER T2 led to 90.37 ± 7.9% expression of the recombined Rosa26 tdTomato reporter in the CD31 + vasculature of the subcutaneous tissue at P4 (Supplementary Fig. 2 ). Recombination outside of the CD31 + vasculature was not detected. Furthermore, we observed only minimal recombination (1.8 ± 0.88%) in iCdh5-tdTomato mice that did not receive tamoxifen (Supplementary Fig. 2 ). To confirm that Gαq hyperactivation in EC induces vascular defects, we additionally employed a Gαq-DREADD mouse (DREADDs are designer receptors exclusively activated by designer drugs) [24] . The DREADD system consists of engineered G protein-coupled receptors (GPCR), which can precisely control GPCR signaling pathways such as Gαq, Gαs or Gαi [24] . Here, we used a Gαq DREADD mouse ( CAG-LSL-Gq-DREADD ) which is a system that expresses a modified M3 muscarinic receptor (hM3Dq) [25] which is only activated upon clozapine-N-oxide (CNO) administration. This mouse line was crossed with Pdgfb-iCreER T2 [16] (hereafter called iPdgfb-hM3Dq ), to induce Gαq activity specifically in EC (Supplementary Fig. 3 ). Injection of tamoxifen on P1 and P2, followed by daily injection of CNO on P3-P8 caused an increase in CD31 + vessel density and vascular area in the skin of iPdgfb-hM3Dq pups at P8 compared to littermate controls (Supplementary Fig. 3 ). Additionally, we analyzed murine brain and retina vasculature. Tufts were detected in the vasculature of both the brain and retina of iPdgfb-GNAQ Q209L mice (Supplementary Fig. 4 , 5 ). Because GNAQ -related vascular anomalies primarily affect capillaries and veins [26] , [27] , [28] , [29] , we sought to determine which type of blood vessels were affected by vascular tuft formation. For this analysis, we utilized the developing vasculature of the retina as a model in which arteries and veins can be readily distinguished [30] . Analysis of mutant iPdgfb-GNAQ Q209L mice at P8 showed that vascular tufts were exclusively localized to retinal veins and capillaries but absent in arteries (Supplementary Fig. 5 ). Endothelial GNAQ Q209L expression in adult mice drives blood vessel dilation and hyperproliferation of EC Here, we wanted to assess if expression of hyperactive GNAQ mutation in the adult vasculature can cause vascular defects. In these studies, we performed tamoxifen injections (two doses of 75 mg/kg) in mice at 6-8 weeks of age. Tissue was harvested one day before 50% of mutant mouse lethality was detected, which corresponded to day 6 after the start of tamoxifen (Fig. 2a ). We did not detect a difference in survival between male and female iCdh5-GNAQ Q209L mutant mice (Supplementary Fig. 6 ). iCdh5-GNAQ Q209L mice developed vascular tufts and aberrant vascular morphogenesis in the subcutaneous tissues of the abdomen (Fig. 2b ). Compared to control mice, the subcutaneous tissue of the iCdh5-GNAQ Q209L mice showed dilated CD31 + vessels, and significant (both p < 0.0001) increase of CD31 + vascular density and vascular area (Fig. 2c ). Furthermore, we analyzed vessel size distribution which revealed increased percentage of large (>100 μm 2 ) vessels in mutant mice compared to controls (Fig. 2d ). Fig. 2: EC-specific GNAQ Q209L expression in adult mice results in increased blood vessel density, abnormal morphogenesis, and EC hyperproliferation. a Schematic describing Tamoxifen regimen for adult mice (6-8 weeks) before experimental analysis of vasculature in subcutaneous and intestinal tissue at day 6 after tamoxifen induction. Kaplan-Meier curve comparing survival percentage of tamoxifen-induced iCdh5-GNAQ Q209L ( n = 28, red) to controls ( n = 20, black, grey, blue). Mouse genotypes are indicated. Gehan–Breslow–Wilcoxon test ( p < 0.0001). b Left panel: Representative low- and high-power photographs of the subcutaneous tissue of tamoxifen-treated iCdh5-GNAQ Q209L and iCdh5 control mouse. Scale bar: 2 mm. Right panel: Representative images of subcutaneous tissue sections immuno-stained for CD31 (dark brown), scale bar: 50μm. c Quantification of vascular density defined as the number of vessels per area and vascular area as percentage of total area. iCdh5-GNAQ Q209L ( n = 17) and control animals ( n = 17). d Vessel size distribution in subcutaneous tissue sections. Percentage of small (<100 µm 2 ) and large (>100 µm 2 ) vessels. e Representative low- and high-power photographs of intestine of tamoxifen-treated iCdh5-GNAQ Q209L and iCdh5 control mouse. Vascular lesions are indicated by red arrowheads. Scale bar: 2 mm. f Representative confocal z-stack images (max. intensity projection) of whole-mount intestinal muscularis stained for CD31 (red). The boxed regions (white dashed lines) are enlarged, and 3D reconstructed. Scale bar: 100 μm. g The intestinal muscularis vasculature was quantified for vessel diameter, vascular area as percentage of total area, tuft number, as well as tuft area normalized to vascular area. iCdh5-GNAQ Q209L (n = 9) and control littermates ( n = 8). h Tamoxifen induction and EdU injection scheme. EdU was administered to iCdh5-GNAQ Q209L and control littermates, 24 h before analysis. i Representative confocal z-stack images (max. intensity projection) of intestinal muscularis whole-mount preparations labeled for EdU (green) and CD31 (red). Images were 3D reconstructed. Scale bar: 20μm. j The number of EdU positive endothelial cells (EdU + /CD31 + ) in iCdh5-GNAQ Q209L ( n = 3) and control littermates ( n = 4) was counted and shown as percentage of total number of endothelial cells (CD31 + ). Data in ( c,g,j ) represented as mean±SD, unpaired two-tailed Welch’s t-test. Mouse genotypes are indicated. Source data for ( a,c,d,g,j ) provided as a Source Data file. Schematic in ( b,e ) created with Biorender.com. Full size image Vascular tufts were also detected in the small intestine of iCdh5-GNAQ Q209L mice at day 6 after tamoxifen induction (Fig. 2e ). Whole-mount CD31 staining of the intestinal muscularis showed that the iCdh5-GNAQ Q209L tissue had significantly ( p < 0.0001) increased vessel diameter, vascular area, and tuft number/area, when compared to the intestinal muscularis of control mice (Fig. 2f, g ). Of note, we generated EC-specific expression of the mutant GNAQ p.Q209L in adult mice with the use of both Cdh5-iCreER T2 and Pdgfb-iCreER T2 and obtained similar phenotypes (Supplementary Fig. 7 ), demonstrating that the observed changes to the vasculature are not dependent on a specific endothelial Cre driver. To test the efficiency and specificity of the Cdh5-iCreER T2 driver in adult mice, we analyzed iCdh5-tdTomato mice. Tamoxifen-induced activation of Cdh5-iCreER T2 in adult mice led to 88.13±2.93% and 91.62±1.12% expression of tdTomato in the CD31 + vasculature in the subcutaneous and intestinal muscularis tissues, respectively (Supplementary Fig. 8 ). We did not detect recombination in non-endothelial cells (CD31 - ). Furthermore, iCdh5-tdTomato mice that did not receive tamoxifen showed only minimal recombination in the subcutaneous and intestinal muscularis tissues (2.7 ± 2.50% and 2.20 ± 1.60%, respectively) (Supplementary Fig. 8 ). Next, we sought to determine if vascular lesions are characterized by increased EC proliferation. To assess the proliferative capacity of EC expressing GNAQ Q209L , we injected mice with EdU (5-Ethynyl-2′-deoxyuridine) to label cells undergoing DNA replication in S phase of the cell cycle. EdU was injected 5 days after tamoxifen induction and mouse tissue was analyzed 24 h after EdU administration (Fig. 2h ). Quantification of EdU + /CD31 + cells in the intestinal muscularis or EdU + /ERG + events in the subcutaneous tissue showed a significantly ( p = 0.0005 and p = 0.0043, respectively) increased number of EdU + EC in iCdh5-GNAQ Q209L mice compared to controls (Fig. 2i, j ; Supplementary Fig. 9 and Movies 3 , 4 ). Increased vascular permeability in iCdh5-GNAQ Q209L mice Vascular lesions in patients, such as pyogenic granulomas, are prone to bleeding [31] . To investigate vascular permeability, we performed whole-mount staining of the intestinal muscularis with CD31 to label the vasculature and TER119 to label the erythrocytes (red blood cells, RBC) in adult mice, 6 days after tamoxifen administration (Fig. 3a, b ). Quantification of extravasated RBC located outside of the CD31 + vascular channels revealed the breakdown of vessel integrity in the iCdh5-GNAQ Q209L mice, while only rare RBC were found outside of the vascular channels in control mice (Fig. 3b, c and Supplementary Movies 5 , 6 ). Fig. 3: EC-specific GNAQ Q209L expression results in vascular hyperpermeability and decreased VE-Cadherin expression. a Tamoxifen induction scheme. b Representative confocal z-stack images of intestinal muscularis whole-mount preparations stained for erythrocytes (TER119 positive cells—white) and CD31 positive endothelium (red). The boxed regions (white dashed lines) are enlarged, 3D reconstructed, and show extravasated TER119 + erythrocytes (yellow arrows). Scale bar: 70 μm. c Quantification of the number of extravasated TER119 + erythrocytes normalized to tissue area. iCdh5-GNAQ Q209L ( n = 9) and control littermates ( n = 8), mean±SD, unpaired two-tailed Welch’s t-test. Mouse genotypes are indicated. d Diagram of experimental procedure for Miles assay. Mice were pretreated with histamine inhibitor followed by intravenous injection of Evans blue dye. This was followed by an intradermal injection of PBS with or without VEGF (100 ng). e Representative photographs of the leakage of Evans Blue dye in dorsal flank skin of iCdh5-GNAQ Q209L and control littermate ( GNAQ Q209L ) that were subjected to Miles assay. Scale bar: 500μm. f Quantification of vascular leakage in the Miles assay. The absorbance (optical density, OD620nm) from each skin sample was normalized to the weight of the tissue sample. iCdh5-GNAQ Q209L ( n = 5) and control littermates ( n = 8), mean±SD, unpaired two-tailed Welch’s t-test. Mouse genotypes are indicated. g Schematic of lentiviral transduction of human endothelial cells. The expression of GNAQ -Q209L or GNAQ -WT was induced by doxycycline (dox) treatment (1 µg/mL). h Immunoblot for VE-Cadherin expression in iEC GNAQ -Q209L or GNAQ -WT after doxycycline treatment for 48 h. Representative of 2 independent experiments. i Representative confocal z-stack images (max. intensity projection) of confluent cell monolayer stained for VE-Cadherin (white). Nuclei were labeled with DAPI (blue). Expression was compared between iEC GNAQ -WT and iEC GNAQ -Q209L upon 1 µg/mL dox treatment. Scale bar: 50μm. j VE-Cadherin positive area was quantified and is shown as percentage of positive area per cell, n = 5 independent experiments per group, mean±SD, unpaired two-tailed Welch’s t-test. Source data for ( c,f,h,j ) are provided as a Source Data file. Schematic in ( b,d,g ) created with Biorender.com. Full size image A previous study demonstrated that EC-specific deletion of GNAQ/11 confers protection against VEGF-A-induced vascular permeability, implicating GNAQ in mediating this process [32] . We thereby hypothesized that hyperactive mutant GNAQ mice would demonstrate enhanced permeability compared to control mice in response to VEGF-A treatment. To analyze the VEGF-A-induced vascular permeability in our iCdh5-GNAQ Q209L mice we performed a Miles assay [33] (Fig. 3d ). We injected Evans Blue dye through the tail vein and assessed blue dye leakage from the vasculature in response to intradermal injection of PBS or VEGF-A. Quantification of the extravasated Evans blue dye revealed increased VEGF-A-induced vascular permeability in the skin of mutant mice compared to controls (Fig. 3e, f ). Endothelial permeability can be regulated by the stability of cell-cell adherens junctions composed by vascular endothelial (VE)-Cadherin [34] . Comparative assessment of VE-Cadherin expression in vivo was not possible because of the stark difference in blood vessel shape and lumen size between mutant and control mice. Thereby, we set out to generate an in vitro model of endothelial GNAQ p.Q209L by transducing endothelial colony-forming cells (ECFC) [35] with lentiviral constructs promoting doxycycline-inducible (i) expression of GNAQ -Q209L or GNAQ -WT (Fig. 3g ). Immunoblotting revealed decreased expression of VE-Cadherin in the mutant iEC GNAQ -Q209L compared to control EC, iEC GNAQ -WT when gene expression was induced by treatment with doxycycline (Fig. 3h ). Furthermore, in confluent cell monolayers, 48 h after doxycycline administration, VE-Cadherin expression at the cell junctions was visibly and significantly ( p = 0.0026) reduced in the mutant EC compared to control GNAQ -WT EC (Fig. 3i, j ). Mice expressing GNAQ Q209L in the vasculature develop thrombocytopenia and severe coagulopathy, mimicking KMP in patients Kasabach-Merritt phenomenon (KMP) is a poorly understood and life-threatening complication of vascular tumors that is characterized by thrombocytopenia and consumptive coagulopathy. KMP may affect up to 70% of all patients with KHE and 10-38% of patients with TA [19] , [36] . To study whether there is a similar complication in our iCdh5-GNAQ Q209L mouse model, we collected blood and performed complete blood counts (CBC) on day 6 after tamoxifen injection (75 mg/kg) (Fig. 4a ). iCdh5-GNAQ Q209L mice showed thrombocytopenia (low number of platelets), with a 42.2% reduction in platelet number compared to control animals. Mutant mice were also anemic, with 35.9% lower red blood cell (RBC) count and 34.5% lower hemoglobin levels, compared to tamoxifen-treated littermates and mutant mice that did not receive tamoxifen (Fig. 4b, c and Supplementary Fig. 10 ). Fig. 4: Mice expressing GNAQ Q209L in the vasculature develop thrombocytopenia and severe coagulopathy. a Tamoxifen induction scheme. b-c Hematological parameters were measured in iCdh5-GNAQ Q209L ( n = 10) and controls ( n = 18), mean±SD, unpaired two-tailed Welch’s t-test. Mouse genotypes are indicated. b Platelet counts, c RBC (red blood cell counts), and hemoglobin levels. d D-Dimer levels were measured in plasma samples from iCdh5-GNAQ Q209L ( n = 23) and controls ( n = 28), mean±SD, unpaired two-tailed Welch’s t-test. Mouse genotypes are indicated. e-f Representative confocal z-stack images (max. intensity projection) of intestinal muscularis stained for e CD41 or f CD42b (red) together with CD31 (green) and TER119 (white/grey). Images are representative of n = 3 mice/group and were 3D reconstructed. Scale bar: 40μm. Source data for ( b,c,d ) are provided as a Source Data file. Schematic in ( e ) created with Biorender.com. Full size image In patients, KMP presents with elevated D-Dimer levels [36] , a marker of fibrin deposition and subsequent fibrinolysis. iCdh5-GNAQ Q209L plasma analysis revealed an average 3.6-fold increase in D-Dimer levels compared with control animals (Fig. 4d ). Prothrombin time (PT) and activated partial thromboplastin time (aPTT) analysis showed that PT was significantly reduced (p = 0.0006) in mutant mice (Supplementary Fig. 11a ). We further analyzed blood smears and quantified polychromasia and schistocytes. Polychromasia was significantly increased (p = 0.0178) in mutant mice compared to tamoxifen-treated control littermates and mutant mice without tamoxifen, while schistocytes were low in all groups (Supplementary Fig. 11b, c ). These data suggest that the anemia was not driven by intravascular hemolysis or red blood cell aplasia. One proposed mechanism for the association of vascular anomalies with systemic thrombocytopenia is the accumulation and sequestration of platelets and fibrin/fibrinogen in the malformed vessels [37] . To assess for platelet accumulation in the vascular tufts, we perfused the mouse prior to tissue collection and stained the intestinal muscularis for CD41 or CD42b, which are markers for platelets. CD41 and CD42b immunostaining was highly enriched in the CD31 + vascular tufts in the mutant iCdh5-GNAQ Q209L mice even upon tissue perfusion, indicating increased adherence to the vessel wall, while being almost absent from perfused control tissue (Fig. 4e, f and Supplementary Movies 7 – 10 ). In the subcutaneous tissue we obtained a similar pattern of platelet localization (Supplementary Fig. 12a–c ). Additionally, we also detected increased fibrin/fibrinogen deposition in the vascular tufts of iCdh5-GNAQ Q209L mice, compared to control mice (Supplementary Fig. 12d ). To determine if hematopoietic alterations also contribute to the systemic thrombocytopenia and anemia, we performed quantitative analysis of the murine hematopoietic stem and progenitor compartments with a 15-fluorochrome flow cytometry protocol [38] , [39] . We did not observe differences in the bone marrow cellularity, the absolute number of hematopoietic stem cell or early multipotent progenitors between the iCdh5-GNAQ Q209L mutant mice and the control mice (Supplementary Fig. 13 ). We detected some subtle variations in the number of late progenitors for the megakaryocytic and erythroid lineages which are most likely associated with compensatory mechanisms to rescue the peripheral thrombocytopenia and anemia. GNAQ p.Q209L expression in endothelial cells drives transcriptional activation of angiogenesis, MAPK signaling, inflammatory response, and coagulation While some effectors of the hyperactive mutant GNAQ p.Q209L have been discovered in the context of uveal melanoma [10] , [40] , [41] , [42] , [43] , [44] , [45] , it is still unclear which EC-specific GNAQ effectors are driving the formation and expansion of vascular abnormalities. To identify the pathways that are modulated by GNAQ p.Q209L expression in EC, we performed transcriptional profiling of human ECFC expressing wild-type (WT) and mutant GNAQ ( n = 4 biological replicates for cell type). The principal component analysis revealed a clear separation between iEC GNAQ -Q209L and iEC GNAQ -WT, indicating significant transcriptional alterations. Importantly, iEC GNAQ -WT with and without doxycycline were similar, showing that GNA Q-WT overexpression has little effect on the transcriptional changes observed in the mutant cells (Fig. 5a ). We found that a total of 917 genes were differentially expressed in iEC GNAQ -Q209L compared to iEC GNAQ -WT, with more up-regulated genes than down-regulated genes (Fig. 5b, c ). KEGG (Kyoto Encyclopedia of Genes and Genomes) and GO-BP (Gene Ontology Biological Pathways) pathway analysis of the differentially expressed genes identified significant changes in multiple pathways (log2 fold change of ≥1.0 or ≤−1.0 and adjusted q-value ≤0.05). Among these, we identified angiogenesis, MAPK signaling, inflammatory response and complement and coagulation pathways (Fig. 5d ). These data were confirmed with Gene Set Enrichment Analysis (GSEA) for the Hallmarks: KRAS signaling up, Angiogenesis, Inflammatory response, TNFα signaling via NFkB, and Complement (Supplementary Fig. 14 ). Furthermore, direct analysis of mRNA expression by qPCR confirmed the modulation of genes in these pathways (Fig. 5e ). Fig. 5: RNA-Sequencing of iEC GNAQ -Q209L reveals enriched expression of genes related to angiogenesis, MAPK signaling, inflammatory response, and coagulation. a Principal Component Analysis (PCA) of RNA-sequencing data obtained from iEC GNAQ -WT no Dox, iEC GN AQ-WT + Dox and iEC GNAQ -Q209L + Dox. b iEC GNAQ -WT and to GNAQ -Q209L (n = 4 biological replicates per group) were treated with 1 µg/mL doxycycline for 24 h and total RNA was collected for RNA-seq analysis. Differentially expressed genes (DEG) are defined as log2 (fold change) ≥1 and adjusted P value of <0.05. Heat maps of differentially expressed transcripts in iEC GNAQ -Q209L compared to GNAQ -WT. Wald test for hypothesis testing. c Volcano-plot of DEGs in iEC GNAQ -Q209L compared to GNAQ- WT. A total of 617 genes showed increased expression while 300 genes showed decreased expression in iEC GNAQ -Q209L compared to iEC GNAQ -WT. d KEGG and GO-BP pathway analyses of DEGs. e A selected group of DEGs were validated using RT-qPCR. n = 4 samples/group ( median and quartiles), unpaired two-tailed Welch’s t-test. f Representative immunoblots of GNAQ, phospho-ERK (pERK, Thr202/Tyr204), total ERK (tERK), phospho-AKT (pAKT, Ser473), total AKT (tAKT), ANGPT2, and GAPDH in iEC GNAQ -WT and GNAQ -Q209L 48 h after doxycycline induction (0, 0.25, 0.5, 1 and 2 μg/ml of Dox). The expression of pERK was quantified and normalized to tERK expression ( n = 3 independent experiments). Mean±SD, one-way ANOVA with Tukey’s multiple comparisons. P-values for statistical analysis between all groups are listed in the Source data file. Source data for ( c,d,e,f ) are provided as a Source Data file. Full size image To validate the upregulation of MAPK signaling and the angiogenic growth factor angiopoietin-2 (ANGPT2) expression at the protein level in the mutant EC expressing GNAQ -Q209L, we performed immunoblotting (Fig. 5f ). Doxycycline administration induced protein expression of GNAQ in a dose-dependent manner in both GNAQ -WT and GNAQ -Q209L expressing cells. Importantly, only mutant iEC GNAQ -Q209L showed increasing and doxycycline dose-dependent levels of activated (phosphorylated) ERK, confirming the MAPK signaling pathway activation, while phosphorylated AKT was not upregulated in the GNAQ mutant EC. ANGPT2 protein expression levels were also increased. Conversely, no ERK activation or ANGPT2 expression were noted in the iEC GNAQ -WT in response to doxycycline administration (Fig. 5f ). Increased endothelial MAPK/ERK signaling in murine and patient-derived tissue expressing GNAQ Q209L To determine that expression of GNAQ Q209L in the vasculature in vivo promotes activation of the MAPK/ERK pathway and increases proliferation we analyzed the subcutaneous tissue of adult mice. The subcutaneous tissue sections were immunostained for ERG to label the EC nuclei, for phospho(p)-ERK and for Ki67 to label cells with increased ERK activation and proliferative capacity, respectively (Fig. 6a, b ). The number of EC per field area was expressed as the number of ERG + cells/mm 2 and was significantly (p = 0.0002) increased in iCdh5-GNAQ Q209L tissue compared to control (Fig. 6c ). The percentage of pERK + ECs and Ki67 + ECs were also significantly (p = 0.0285 and p = 0.0185) increased. There was also a trend of increased number of double-positive pERK + /Ki67 + ECs in the iCdh5-GNAQ Q209L tissues compared to controls (Fig. 6c ). Fig. 6: Increased ERK activation in the vasculature of GNAQ Q209L expressing mice and patient vascular tumor. a Tamoxifen induction scheme for analysis of subcutaneous tissue. b Representative images of subcutaneous tissue of tamoxifen-treated control and iCdh5-GNAQ Q209L mutant mice stained for ERG (white), pERK (red), Ki67 (green), and merge. Scale bar: 50 μm. c ERG staining marks EC nuclei. Quantification of ERG + cells normalized per subcutaneous tissue area. pERK + and Ki67 + and double-positive endothelial cells were normalized to total EC number. iCdh5-GNAQ Q209L ( n = 9) and control littermates ( n = 9), mean±SD, unpaired two-tailed Welch’s t-test. Mouse genotypes are indicated. d GNAQ Q209L mutant patient-derived vascular tumor tissue was analyzed. e Representative images of neonatal human foreskin and patient-derived tissue (cutaneous vascular tumor) with somatic GNAQ p.Q209L mutation immuo-stained for UEAI (Ulex europaeus agglutinin-I) (brown). Scale bar: 50μm. f Representative images of neonatal human foreskin and patient-derived tissue with somatic GNAQ p.Q209L mutation labeled for UEAI (white), pERK (red), Ki67 (green), and merge with DAPI (blue). Scale bar: 50 μm. g Quantification of the UEAI + vascular area as percentage of total field area, pERK + , Ki67 + and double-positive EC calculated as events per mm 2 of vascular area; human foreskin tissue from n = 5 different donors, and n = 1 patient-derived tumor tissue, mean±SD. Source data for ( c,g ) are provided as a Source Data file. Schematic in ( a,d ) created with Biorender.com. Full size image To confirm the relevance of these results, we also analyzed a patient-derived cutaneous vascular tumor with a somatic GNAQ p.Q209L mutation (Fig. 6d ). The tumor tissue showed numerous blood vessels and tufts of EC as shown by staining with the human-specific endothelial lectin Ulex Europaeus Agglutinin-I (UEAI) (Fig. 6e ). The patient tissue was compared to control human neonatal foreskin from 5 different donors. Quantification of the UEAI + vascular area showed that it was increased in the lesional patient tissue compared to normal foreskin (Fig. 6f, g ). Furthermore, the number of pERK + ECs, Ki67 + ECs and double-positive (pERK + /Ki67 + ) ECs were higher in the patient tissue compared to control human foreskin from 5 different donors (Fig. 6g ). Trametinib treatment rescues vascular phenotype, EC hyperproliferation, thrombocytopenia, and prolongs survival of GNAQ mutant mice To investigate the role of Gαq downstream effector MAPK/ERK in the pathogenesis of vascular anomalies in our GNAQ Q209L mouse model, we performed proof-of-concept experiments with the MEK/ERK inhibitor, Trametinib (MEKINIST®). First, we tested the efficacy of Trametinib in a preventative scheme. We performed tamoxifen injections (2 daily doses of 75 mg/kg) in 6-week-old iCdh5-GNAQ Q209L mutant mice, while also delivering Trametinib (2 mg/kg) or vehicle, once daily (Fig. 7a ). On day 5 (corresponding to 90% survival rate of mutant iCdh5-GNAQ Q209L mice), tissues were harvested. To evaluate the ability of Trametinib to antagonize the development of vascular anomalies, subcutaneous tissue and intestinal muscularis were analyzed. Macroscopic images and CD31 immunostaining revealed decreased vascularity in the subcutaneous tissue sections of Trametinib-treated mutant mice compared to vehicle-treated mice. (Fig. 7b ). Trametinib-treated mutant mice showed reduced percentage of large vessels (15.4 ± 3.4%) compared to vehicle-treated (25.7 ± 7.3%) mutant mice (Fig. 7c ) and reduced vascular density and vascular area, which reached values similar to unchallenged control mice (see dotted lines) (Fig. 7d ). Fig. 7: Trametinib treatment of GNAQ Q209L mutant mice rescues vascular phenotype, hyperproliferation, permeability and coagulopathy. a Preventative study scheme. 6 weeks-old iCdh5-GNAQ Q209L mice induced with 75 mg/kg tamoxifen and concomitantly treated with Trametinib (2 mg/kg/day) or vehicle. b Macroscopic photographs of subcutaneous tissue from vehicle and Trametinib -treated mice. CD31 (dark brown) stained tissue sections. Scale bars: 2 mm and 50μm. c Vessel size distribution in subcutaneous tissue as percentage of small (<100 µm 2 ) and large (>100 µm 2 ) vessels. d Vascular density and area in vehicle or Trametinib -treated mice. e Representative photograph of intestine from vehicle and Trametinib -treated iCdh5-GNAQ Q209L mice. Whole-mount intestinal muscularis stained for CD31 (red), z-stack maximum intensity projection. Scale bars: 2 mm and 100 μm. f Quantification of intestinal muscularis vessel diameter, vascular area, tuft number and tuft area. g Intestinal whole-mounts labeled for EdU (green) and CD31 (red). Scale bar: 20μm. h EdU positive EC (EdU + /CD31 + ) as percentage over total EC number (CD31 + ). i Representative z-stack maximum intensity projection of intestinal muscularis stained for TER119 (white) and CD31 (red). Yellow arrows indicate extravasated erythrocytes. Scale bar: 100μm. j Quantification of extravasated erythrocytes normalized to tissue area. k Platelet counts and D-Dimer levels in vehicle or Trametinib -treated iCdh5-GNAQ Q209L mice. In d , f , h , j and k : vehicle ( n = 7), Trametinib (n = 8), mean±SD, unpaired two-tailed Welch’s t-test. Black dotted lines indicate reference values in untreated control mice. l Representative immunoblot of iEC GNAQ -Q209L treated with DMSO or Trametinib and probed for GNAQ, phosphor-ERK (pERK, Thr202/Tyr204), total ERK (tERK), and GAPDH ( n = 3 independent experiments). m Venn diagram of genes upregulated in iEC GNAQ -Q209L and downregulated with Trametinib treatment (6 h). Expression levels of 73 genes were normalized by Trametinib (adjusted P -value of <0.05 and a log2 (fold change) >1). Heatmap of selected genes clustered by GO-terms. Wald test for hypothesis testing. n Therapeutic study scheme. 6 weeks-old iCdh5-GNAQ Q209L mice induced with 40 mg/kg tamoxifen and after 8 days treated daily with Trametinib (2 mg/kg) or vehicle. Kaplan-Meier survival curve of vehicle ( n = 8, red) and Trametinib -treated ( n = 9, turquoise) iCdh5-GNAQ Q209L mice. Gehan-Breslow-Wilcoxon test. Trametinib-treated control mice ( iCdh5 mice, n = 3, blue). Source data for ( c,d,f,h,j,k,l,m,n ) are provided as a Source Data file. Schematic in ( b,e ) created with Biorender.com. Full size image Intestinal muscularis was analyzed macroscopically and by whole-mount immunofluorescence CD31 staining (Fig. 7e ). Trametinib treatment normalized CD31 + vessel diameter and vascular area compared to vehicle-treated iCdh5-GNAQ Q209L mice (Fig. 7f ). Furthermore, the Trametinib-treated mice showed a significant ( p = 0.0082 and p < 0.0001) reduction in the number of tufts, as well as tuft area (Fig. 7f ). To determine if Trametinib affects the proliferative capacity of EC in the mutant mice, we injected mice with EdU 24 h before the analysis at day 5 (see schematic in Fig. 7a ). Quantification for EdU + /CD31 + events showed a significant ( p < 0.0001) decrease in the number of EdU + EC in the intestinal muscularis (Fig. 7g, h and Supplementary Movies 11 , 12 ) and in the subcutaneous tissue of Trametinib-treated iCdh5-GNAQ Q209L mice compared to vehicle-treated (Supplementary Fig. 15 ). Trametinib treatment additionally rescued the vascular permeability of iCdh5-GNAQ Q209L mice (Fig. 7i ). The number of extravasated TER119 + erythrocytes was significantly reduced ( p = 0.0036) in Trametinib-treated mice compared to vehicle-treated and reached values similar to unchallenged control mice (Fig. 7j ). Furthermore, blood cell analysis revealed a rescue of the platelet number in the Trametinib-treated iCdh5-GNAQ Q209L mice (Fig. 7k , Supplementary Fig. 16 ), reaching comparable levels to unchallenged control mice (see dotted line) and significantly ( p = 0.0386) higher than vehicle-treated mice. Plasma analysis showed that D-Dimer levels were significantly ( p = 0.0086) lower in Trametinib-treated iCdh5-GNAQ Q209L mice, thereby Trametinib prevented the onset of coagulopathy (Fig. 7k ). The efficacy of Trametinib in inhibiting the MAPK/ERK pathway in iEC GNAQ -Q209L was confirmed by immunoblotting. Treatment of iEC GNAQ-Q209L with Trametinib (1 and 5 nM) for 24 h suppressed ERK activation in a dose-dependent manner (Fig. 7l ). Next, to identify the MEK-dependent targets of hyperactive mutant GNAQ , we performed transcriptional profiling in iEC GNAQ -Q209L treated with Trametinib or vehicle and compared them to vehicle-treated iEC GNAQ -WT control cells (Fig. 7m ). We identified 617 genes whose expression was upregulated in iEC GNAQ -Q209L compared to iEC GNAQ -WT. The expression levels of 73 of these genes were restored to normal levels in response to Trametinib treatment. Among these we identified genes implicated in the MAPK pathway activity, inflammatory response and Notch signaling (Fig. 7m ). GSEA revealed that Trametinib treatment resulted in the normalization of upregulated genes associated with hallmark gene signatures of KRAS Signaling Up, Angiogenesis, TNFα signaling via NFkB, Inflammatory response, Complement, and Coagulation (Supplementary Fig. 17 ). Lastly, we performed pre-clinical treatment studies to determine the therapeutic efficacy of Trametinib in promoting the survival of mutant mice. For these studies we used a lower dose of tamoxifen (40 mg/kg) which resulted in 50% lethality at day 13-15 (Supplementary Fig. 18 ). Daily Trametinib treatment started 8 days after tamoxifen induction, and significantly ( p = 0.0014) extended the life span of the mutant mice of up to 9 days compared to the vehicle-treated mice (Fig. 7n ). Vehicle or Trametinib treatment of genetic controls did not result in illness or morbidity. Somatic mutations in GNAQ/11/14 that cause gain-of-function constitutively active Gαq signaling have been identified in a variety of vascular anomalies, including malformations and tumors. Despite these findings, genetic animal models for Gαq driven vascular anomalies have not yet been reported. Therefore, the cellular and molecular determinants of constitutively active GNAQ signaling in blood vessel dysmorphogenesis have not been investigated. In this study, we generated a murine model of mutant GNAQ -driven vascular tumors by conditionally expressing GNAQ Q209L in Cdh5 (or Pdgfb ) expressing ECs. This model recapitulated common histopathological findings in vascular tumors with GNAQ/11/14 mutations. These include the formation of vascular tufts which are lobules of proliferative and irregularly structured vascular lesions. Vascular tufts in mutant mice were characterized by hyperproliferation and increased permeability. Furthermore, our GNAQ Q209L mouse model developed a coagulopathy that resembles KMP, a life-threatening coagulopathy seen in some of these patients. Lastly, we investigated the transcriptomic effects of GNAQ Q209L signaling and determined that angiogenesis, MAPK/ERK signaling, coagulation and inflammation pathways are increased. In proof-of-concept studies, we showed that Trametinib, a MEK/ERK inhibitor, rescues the aberrant vascular morphogenesis, hyperproliferation, permeability, KMP-like coagulopathy, and extended mutant mouse survival, suggesting that MAPK/ERK signaling drives these phenotypic manifestations. Our murine model was generated with the use of inducible EC-specific Cre-drivers to study the effects of constitutively active GNAQ in the endothelium. In patients, GNAQ/11/14 mutations are somatic ( i.e ., non-inherited) and the allelic frequency in the patients’ affected tissue is generally quite low. Studies in congenital hemangioma and capillary malformation reported enrichment of the GNAQ mutation in the EC population, strongly suggesting the mutations originate in EC [1] , [46] , [47] . To drive expression of GNAQ Q209L in EC we used Cdh5-iCreER T2 or Pdgfb-iCreER T2 Cre driver murine lines. It is worth noting that we did not detect major phenotypical differences between iCdh5-GNAQ Q209L and iPdgfb-GNAQ Q209L animals. The presence of somatic activating GNAQ mutations in vascular anomalies suggests an essential role for Gαq signaling in vascular development and homeostasis. Here, we show that the GNAQ mutation p.Q209L is sufficient for the formation of hyperproliferative vascular lesions when driven solely in EC. Previous studies have shown that deficiency of Gαq and/or Gα11 in endothelial cells resulted in reduced EC proliferation and impaired retinal angiogenesis, while conferring protection against VEGF-A-induced vascular permeability [32] . In our study we further demonstrate the essential role of GNAQ in vascular permeability and show that gain-of-function GNAQ mutations can promote vascular leakage and disrupt VE-Cadherin expression in adherens junctions. Taken together, this demonstrates that both gain-of-function and loss-of-function GNAQ mutations can result in abnormal angiogenesis. GNAQ/11 gain-of-function mutations are very frequent in uveal melanoma, an aggressive tumor of melanocytes in the uveal tract of the eye. In this context, it has been found that GNAQ Q209L can lead to hyperactivation of the downstream MAPK/ERK signaling pathway as well as activation of the Hippo pathway through nuclear localization of YAP1 via a Trio-Rho/Rac signaling circuit [11] . To date, MAPK inhibitors have not shown clinical benefit for uveal melanoma patients, making the role of MAPK in uveal melanoma less clear. In fact, many studies rely on poorly characterized melanoma cell lines that express multiple mutation types [48] , [49] , while studies with primary uveal melanomas reported very heterogeneous levels of ERK activation, suggesting there is no association with GNAQ/11 mutations [50] , [51] . In our studies, we generated transcriptomic data to show that MAPK and KRAS pathways are among the most upregulated signaling pathways in EC expressing GNAQ Q209L . We also went on to confirm increased pERK levels in tissues of our iCdh5-GNAQ Q209L animal model and in a patient-derived vascular tumor tissue with a confirmed somatic GNAQ p.Q209L mutation. Although different GNAQ mutations are associated with different classes of vascular anomalies (such as GNAQ R183Q and GNAQ Q209R in CM and GNAQ Q209L in vascular tumors), recent studies highlighted that the transcriptional consequences of these mutations in ECs are similar and include upregulation of pathways such as MAPK, angiogenesis, inflammation via TNFα and NFkB, and upregulation of ANGPT2 [12] , [52] . Published data also suggest that the differences between these GNAQ mutation types affect the level of activation/expression rather than the specific downstream targets [12] . Furthermore, similar to a recent study in melanocytes, we did not detect significant upregulation of genes associated with the non-canonical activation of the Hippo pathway [42] . To date, only few direct inhibitors of Gαq/11 have been reported. Among these are YM-254890 and FR900359, which are natural products isolated from the bacterium Chromobacterium and from the plant Ardisia crenata Sims . While these compounds showed efficacy in inhibiting abnormal signaling in Gαq mutant uveal melanoma cell lines, their complex chemical structures have hindered their commercial development [41] , [53] , [54] . For this reason, additional pathways and effectors have been investigated and shown to be important for uveal melanoma tumorigenesis such as PKC, Trio/Rho/Rac, YAP/TAZ, and FAK [44] , [55] , [56] . Several studies have shown the efficacy of mono- or -dual therapy in laboratory models. However, targeted therapy in patients is still an unmet clinical need. While the role of these effectors has not yet been explored in GNAQ -related vascular anomalies, our results show that MEK/ERK inhibition with Trametinib in the murine model prevented vascular lesions and the associated complications such as coagulopathy, suggesting this pathway is implicated in the disease pathogenesis. Recently published reports have shown that the hyperactive RAS/MAPK signaling is implicated in other vascular tumors and malformations [57] and some authors successfully modeled mouse vascular anomalies associated with KRAS-G12D/V activating mutations [58] , [59] , [60] . These models showed improvement of the vascular phenotype upon treatment with Trametinib. Clearly, RAS/MAPK signaling is implicated in the manifestation of vascular anomalies, and as such it will be a critical area for future drug development. However, it is important to notice that in our study, while Trametinib treatment significantly improved survival compared to vehicle treatment, mice failed to thrive beyond day 18. In vascular anomalies, this could be explained by the activity of MAPK-independent pathways downstream of the mutant GNAQ . Among the 617 genes upregulated in the EC expressing GNAQ -Q209L, Trametinib treatment normalized the expression of 73 genes, but 544 remained elevated. Future studies should focus on these genes for the identification of targets that could be used in combination with MEK/ERK inhibition to increase therapeutic efficacy. KMP is a life-threatening complication with high morbidity and mortality up to 30% [17] , [19] . Death usually occurs from life-threatening hemorrhage or cardiac failure. KMP affects patients with KHE and TA [19] , [36] , and is characterized by severe thrombocytopenia and consumptive coagulopathy. While the discovery of GNAQ/11/14 mutations in vascular anomalies is recent, a few studies have already reported an association between KMP and gain-of-function GNA11 or GNA14 mutations in patients [3] , [27] . To date, no murine models have been described that replicate the clinical characteristics of KMP, preventing investigation of the cellular and molecular mechanisms regulating the development of this coagulopathy. As a consequence, there is only one proposed cellular mechanism for the association of vascular anomalies with thrombocytopenia, which is the trapping of platelets in malformed vessels [37] . Our iCdh5-GNAQ Q209L model recapitulates several important features of KMP such as thrombocytopenia, anemia, elevated D-dimer, and accumulation of platelets and fibrinogen in vascular tufts. This local trapping of platelets and fibrinogen consumption could lead to increased risk of bleeding. Our study phenocopied important aspects of GNAQ -related vascular tumors and suggests that treatment with MEK/ERK inhibitors could prevent or slow the onset of coagulopathy. EC are crucially involved in vascular hemostasis. In fact, EC maintain blood fluidity by providing an anticoagulant and antithrombogenic boundary layer and by producing regulators of platelet activity. In our transcriptomic data in EC, we showed that coagulation and complement pathways were among the top differentially expressed gene sets in cultured iEC GNAQ -Q209L compared to iEC GNAQ -WT. These findings strongly suggest that transcriptional changes within the mutant GNAQ EC could be driving the hemostatic changes associated with KMP. By transcriptomic analysis, we have also shown that Trametinib can restore the upregulation of genes implicated in complement and coagulation directly on the ECs. Trametinib can also inhibit platelet MEK making it plausible that KMP resolution is facilitated by a dual effect on EC and platelets [61] . However, further studies are needed to dissect the cell-specific effects of Trametinib on KMP. Finally, our study also has a few limitations. 1. Here we used mutant GNAQ Q209L to model common pathological features in tumors with GNA -Q, −11, and −14 hyperactive mutations. While these Gαq gene family members share about 90% sequence homology, future investigations could uncover phenotypical and signaling differences related to the specific mutated gene. 2. While in patients, lesions are visible and often disfiguring, in our murine models they could be detected only after dissection. Measurable superficial skin lesions did not form presumably because widespread vascular defects caused early lethality. For this reason, we used the subcutaneous and intestinal muscle tissue as model tissues to evaluate changes in the vasculature before a superficial visible lesion formed. Future studies should focus on local tamoxifen delivery to better mimic the somatic nature of the events occurring in patients. Furthermore, different doses of tamoxifen could be used to vary the number of cells that undergo CreER T2 -mediated recombination and turn on GNAQ Q209L expression, influencing the severity of the resulting phenotype. 3. In addition, as discussed above, while we expect MAPK/ERK to be an important determinant of the vascular phenotypes (hyperproliferation and vascular permeability), our results do not exclude the involvement of other important pathways. In conclusion, our results confirm that GNAQ plays an essential role in vascular development and homeostasis. The study of its mutations and molecular interactions is of great interest because it may provide new therapeutic targets to prevent the progression of vascular anomalies as well as the potentially lethal complication of KMP. The model we report here should be instrumental for testing novel targeted therapeutic strategies for the treatment of patients affected by GNAQ -related vascular tumors. Mouse models Mice were cared for in accordance with the National Institutes of Health guidelines, and all procedures have been reviewed and approved by the CCHMC Institutional Animal Care and Use Committee (Protocol number IACUC 2020-0039). To study the effects of constitutive active GNAQ expression in the developing and adult vasculature, we utilized different breeding strategies. Both male and female mice were included in the study. CMV-Cre; GNAQ Q209L mice (CMV-GNAQ Q209L ) We examined the effects of GNAQ Q209L expression during embryonic development by crossing the Rosa26-floxed stop-GNAQ Q209L [13] mice with the ubiquitously expressed CMV-Cre (Jax stock No: 006054) [14] . Offspring (postnatal) and embryos (E.8.5 and E.13.5) were genotyped and Mendelian ratios were calculated. Cdh5-iCreER T2 ; GNAQ Q209L mice (iCdh5-GNAQ Q209L ) The endothelial-specific, tamoxifen-inducible Cre-driver line Cdh5 (PAC)-iCreER T2 [15] ( iCdh5 ) was crossed with the Rosa26-floxed stop-GNAQ Q209L ( Gt(ROSA)26Sor tm1(GNAQ*)Cvr [13] ) mouse ( GNAQ Q209L ). Pups received intragastric tamoxifen injection at P1 (10 µg). Adult mice (6-8 weeks) received 75 mg/kg or 40 mg/kg of tamoxifen intraperitoneally (i.p.). Tamoxifen-injected littermates (genotype: WT , Cdh5-iCreER T2 , GNAQ Q209L ) and no-tamoxifen mutant mice were used as controls. The vascular phenotype was analyzed for vascular abnormalities in subcutaneous tissue and intestinal muscularis . Pdgfb-iCreER T2 ; GNAQ Q209L mice (iPdgfb-GNAQ Q209L ) Pdgfb-iCreER T2 is a widely used transgenic mouse line that expresses a tamoxifen-inducible form of Cre-recombinase (iCreER T2 ) [16] in endothelial cells. Pdgfb-iCreER T2 [16] mice were crossed with the Rosa26-floxed stop-GNAQ Q209L mouse. Pregnant dams received tamoxifen i.p. 15 mg/kg and/or pups received intragastric tamoxifen injection at P1 (1 µg). Adult mice (6-8 weeks) received 75 mg/kg of tamoxifen i.p.. Tamoxifen-injected littermates (genotype: WT , Pdgfb-iCreER T2 , GNAQ Q209L ) were used as controls. The vascular phenotype was analyzed for vascular abnormalities in brain, retina, subcutaneous tissue and intestinal muscularis . Pdgfb-iCreER T2 ; hM3Dq mice (iPdgfb-hM3Dq) We used Gαq-DREADD mouse [24] that expresses a modified M3 muscarinic receptor (hM3Dq) [25] . This mouse line, CAG-LSL-Gq-DREADD (Jax Stock No: 026220) [25] was crossed with Pdgfb-iCreER T2 [16] , to induce Gαq activity specifically in the endothelial cells (EC). Pups were injected with tamoxifen (10μg) at postnatal day 1 and 2 and with CNO (5μg/g) daily from P3-P8. The vascular phenotype was analyzed for vascular abnormalities in the skin. Cdh5-iCreER T2 ; Tdtomato mice (iCdh5-tdTomato) The Rosa26-floxed stop-tdTomato reporter mouse was crossed with Cdh5-iCreER T2 to generate a mouse with EC-specific tdTomato expression ( iCdh5-tdTomato ). Pups received intragastric tamoxifen injections at P1 (10μg) and subcutaneous tissue was analyzed at P4. Adult mice (6-8 weeks) were tamoxifen injected (i.p. 75 mg/kg) on 2 subsequent days and analyzed at day 6 after first tamoxifen injection for vascular phenotype in subcutaneous and intestinal muscularis tissue. Whole-mount staining and tissue sections were analyzed for CD31 and tdTomato expression. iCdh5-tdTomato mice injected with sunflower oil only (no tamoxifen) were used as controls. Mouse husbandry Mice were housed in the animal care facility of CCHMC under standard pathogen-free conditions with a 14 h light/10 h dark schedule and provided with food (LabDiet, #5010) and water ad libitum, temperature 22 °C and ~40% relative humidity. All mice were maintained on a C57BL/6 background and both male and female mice were used in all experiments. For survival studies of iCdh5-GNAQ Q209L mice (75 mg/kg or 40 mg/kg of tamoxifen schemes) female and male mice data was analyzed separately and did not show significant differences between the two groups. Therefore, in subsequent studies, data from female and male mice were pooled together. Mice were genotyped using EconoTaq Plus green 2X Master Mix (Lucigen). 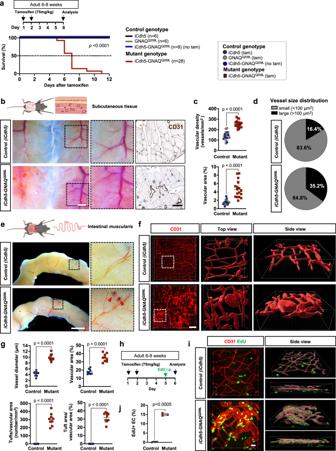Fig. 2: EC-specificGNAQQ209Lexpression in adult mice results in increased blood vessel density, abnormal morphogenesis, and EC hyperproliferation. aSchematic describing Tamoxifen regimen for adult mice (6-8 weeks) before experimental analysis of vasculature in subcutaneous and intestinal tissue at day 6 after tamoxifen induction. Kaplan-Meier curve comparing survival percentage of tamoxifen-inducediCdh5-GNAQQ209L(n= 28, red) to controls (n= 20, black, grey, blue). Mouse genotypes are indicated. Gehan–Breslow–Wilcoxon test (p< 0.0001).bLeft panel: Representative low- and high-power photographs of the subcutaneous tissue of tamoxifen-treatediCdh5-GNAQQ209LandiCdh5control mouse. Scale bar: 2 mm. Right panel: Representative images of subcutaneous tissue sections immuno-stained for CD31 (dark brown), scale bar: 50μm.cQuantification of vascular density defined as the number of vessels per area and vascular area as percentage of total area.iCdh5-GNAQQ209L(n= 17) and control animals (n= 17).dVessel size distribution in subcutaneous tissue sections. Percentage of small (<100 µm2) and large (>100 µm2) vessels.eRepresentative low- and high-power photographs of intestine of tamoxifen-treatediCdh5-GNAQQ209LandiCdh5control mouse. Vascular lesions are indicated by red arrowheads. Scale bar: 2 mm.fRepresentative confocal z-stack images (max. intensity projection) of whole-mount intestinalmuscularisstained for CD31 (red). The boxed regions (white dashed lines) are enlarged, and 3D reconstructed. Scale bar: 100 μm.gThe intestinalmuscularisvasculature was quantified for vessel diameter, vascular area as percentage of total area, tuft number, as well as tuft area normalized to vascular area.iCdh5-GNAQQ209L(n = 9) and control littermates (n= 8).hTamoxifen induction and EdU injection scheme. EdU was administered toiCdh5-GNAQQ209Land control littermates, 24 h before analysis.iRepresentative confocal z-stack images (max. intensity projection) of intestinalmusculariswhole-mount preparations labeled for EdU (green) and CD31 (red). Images were 3D reconstructed. Scale bar: 20μm.jThe number of EdU positive endothelial cells (EdU+/CD31+) iniCdh5-GNAQQ209L(n= 3) and control littermates (n= 4) was counted and shown as percentage of total number of endothelial cells (CD31+). Data in (c,g,j) represented as mean±SD, unpaired two-tailed Welch’s t-test. Mouse genotypes are indicated. Source data for (a,c,d,g,j) provided as a Source Data file. Schematic in (b,e) created with Biorender.com. Genotyping primers are indicated in Supplementary Table 2 . Birth was defined as postnatal day 0 (P0). The Cre-LoxP system was activated through tamoxifen (dissolved in sunflower oil) injections. All animals were monitored once a day for changes in their health conditions. According to guidelines established in our IACUC protocol, mice were humanely euthanized upon signs of moribundity, including lethargy, respiratory distress, and neurological defects. For endpoint studies, mice were euthanized at the established timepoint by carbon dioxide inhalation and cervical dislocation. For studies in which mice were perfused prior to tissue collection, anesthetized mice were perfused transcardially with HBSS through the left ventricle for 10 min. Macroscopic images of subcutaneous and intestinal tissues were taken with a Leica S8 APO stereomicroscope equipped with a Flexacam C3 camera (Leica). The specific MEK1/2 inhibitor Trametinib (GGSK-1120212, LC laboratories, cat#T8123) was dissolved in DMSO (5 mg/mL, Sigma, Cat# D8418). Vehicle solutions for oral dosing were prepared by adding Polyethylene glycol 300 (4 mL, Sigma, cat# 807484), Tween 80 (0.5 mL, Fisher Scientific, cat# BP338-500), and normal saline (14.5 mL, Baxter, cat#2F7124). Mice were administered vehicle or Trametinib (2 mg/kg) via daily gavage. Patient tissue samples The study was performed in accordance with the Declaration of Helsinki, and the patient tissue sample was obtained after written informed consent. This study used samples, data, and/or services from the Discover Together Biobank at Cincinnati Children’s Research Foundation. All the procedures were approved by the Institutional Review Board according to ethical guidelines (Approved IRB # 2016-3878 and # 2017-3726 per institutional policies) at Cincinnati Children’s Hospital Medical Center (CCHMC), with approval of the Committee on Clinical Investigation. Samples were obtained without identifiers and include excised tumor tissue sections and neonatal foreskin for immunohistochemistry and immunofluorescent staining. We do not have information on the sex/gender of the human subject of the tumor sample in the study as the specimen was deidentified. Neonatal foreskin is routinely collected from newborn males. Immunohistochemistry of paraffin-embedded tissue Patient-derived tumor tissue and subcutaneous tissue and muscle of the abdomen of adult mice was fixed in 4% paraformaldehyde (PFA, Electron microscopy Sciences, cat#15710), embedded in paraffin, and sectioned at 5 μm for staining. Slides were deparaffinized with xylene and rehydrated through a descending ethanol series. Antigen retrieval was performed by boiling the slides in 0.01 M citric acid (pH 6.0). Slides were blocked overnight at 4 °C using 5% bovine serum albumin (BSA, Sigma, cat#A7906) in 0.1 M phosphate buffer saline (PBS, Fisher Scientific, cat#BP3994) containing 0.3% Triton X-100 (Sigma, cat#X100). To visualize vasculature, mouse tissue specimens were incubated overnight with the following primary antibodies: rabbit anti-CD31 (Cell Signaling, cat#77699, clone D8V9E, 0.062 µg/mL) or rabbit anti-mouse fibrinogen antiserum [62] , followed by incubation with biotinylated anti-rabbit antibody (Vector laboratories, cat#BA-1000, 7.5 µg/mL) at RT for 2 h. Human specimens were incubated with biotinylated UEA-I (Vector laboratories, cat#B-1065-2, 20 µg/mL) diluted in PBS containing 5% BSA for 1 h at room temperature (RT). Peroxidase was quenched using 3% hydrogen peroxide H 2 O 2 (Sigma, cat#H1009), followed by a 2 h incubation at RT with Horseradish Peroxidase (HRP) Streptavidin (Vector laboratories, cat#SA-5004-1, 5 µg/mL) and diaminobenzidine (DAB) (Vector laboratories, cat#SK-4100). The slides were counterstained with hematoxylin (Vector laboratories, cat#H-3401-500). For vascular area and vascular density analysis eight high-power field images (20x) were taken randomly per section using Nikon Eclipse CiS microscope, followed by vascular density (vessels/mm 2 ) and vascular area (%) quantification with FIJI software (v1.54b, National Institutes of Health (NIH), Bethesda) [63] . 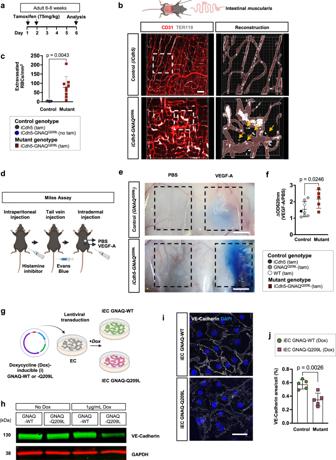Fig. 3: EC-specificGNAQQ209Lexpression results in vascular hyperpermeability and decreased VE-Cadherin expression. aTamoxifen induction scheme.bRepresentative confocal z-stack images of intestinalmusculariswhole-mount preparations stained for erythrocytes (TER119 positive cells—white) and CD31 positive endothelium (red). The boxed regions (white dashed lines) are enlarged, 3D reconstructed, and show extravasated TER119+erythrocytes (yellow arrows). Scale bar: 70 μm.cQuantification of the number of extravasated TER119+erythrocytes normalized to tissue area.iCdh5-GNAQQ209L(n= 9) and control littermates (n= 8), mean±SD, unpaired two-tailed Welch’s t-test. Mouse genotypes are indicated.dDiagram of experimental procedure for Miles assay. Mice were pretreated with histamine inhibitor followed by intravenous injection of Evans blue dye. This was followed by an intradermal injection of PBS with or without VEGF (100 ng).eRepresentative photographs of the leakage of Evans Blue dye in dorsal flank skin ofiCdh5-GNAQQ209Land control littermate (GNAQQ209L) that were subjected to Miles assay. Scale bar: 500μm.fQuantification of vascular leakage in the Miles assay. The absorbance (optical density, OD620nm) from each skin sample was normalized to the weight of the tissue sample.iCdh5-GNAQQ209L(n= 5) and control littermates (n= 8), mean±SD, unpaired two-tailed Welch’s t-test. Mouse genotypes are indicated.gSchematic of lentiviral transduction of human endothelial cells. The expression ofGNAQ-Q209L orGNAQ-WT was induced by doxycycline (dox) treatment (1 µg/mL).hImmunoblot for VE-Cadherin expression in iECGNAQ-Q209L orGNAQ-WT after doxycycline treatment for 48 h. Representative of 2 independent experiments.iRepresentative confocal z-stack images (max. intensity projection) of confluent cell monolayer stained for VE-Cadherin (white). Nuclei were labeled with DAPI (blue). Expression was compared between iECGNAQ-WT and iECGNAQ-Q209L upon 1 µg/mL dox treatment. Scale bar: 50μm.jVE-Cadherin positive area was quantified and is shown as percentage of positive area per cell,n= 5 independent experiments per group, mean±SD, unpaired two-tailed Welch’s t-test. Source data for (c,f,h,j) are provided as a Source Data file. Schematic in (b,d,g) created with Biorender.com. Further antibody details are listed in Supplementary Table 3 . Immunofluorescent staining and quantification of tissue sections For immunofluorescent triple labeling, sections were blocked using 5% BSA in PBS containing 0.5% Triton X-100 overnight at 4 °C. Next, specimens were incubated with rabbit anti-pERK 1/2 (Phospho-p44/42 MAPK Thr202/Tyr204, Cell signaling, cat#9101, 5 µg/mL) antibody at 4 °C overnight. Subsequently, sections were incubated for 2 h at RT with a biotinylated anti-rabbit antibody (Vector laboratories, cat#BA-1000, 7.5 µg/mL) and Texas Red® Streptavidin (Vector laboratories, cat#SA-5006-1, 5 µg/mL) for 2 h at RT. Next, sections were incubated with Alexa Fluor TM 488 conjugated (A488) anti-Ki67 (Cell Signaling, cat#11882, clone D3B5, 2 µg/mL) overnight at 4 °C. Subsequently, slides were incubated with anti-ERG-A647 (Abcam, cat#ab196149, clone EPR3864, 5 µg/mL, mouse) or UEA-I DyLight TM 649 (Vector laboratories, cat#DL-1068-1, 20 µg/mL, human), at 4 °C overnight and counterstained with 4’,6-Diamidino-2-Phenylindole, Dihydrochloride (DAPI, cat#D1306, Invitrogen, 5 µg/mL) for 5 min at RT. Sections were mounted with Fluoromount-G® mounting medium (Southern Biotech, cat#0100-01). For quantitative analysis of mouse tissues, five randomly assigned regions were imaged per section using Nikon Eclipse T1 microscope. Image analysis and quantification were performed using the open-source software CellProfiler [64] . A CellProfiler pipeline was designed to detect and count ERG, pERK and Ki67-positive cells from immunofluorescence images using automatic thresholding and segmentation methods. For mouse tissue, cells identified as double or triple positive were quantified and expressed as percentage of the number of ERG-positive EC. For quantitative analysis of patient-derived tissue, 5-11 randomly assigned regions were imaged per section using Nikon Eclipse T1 microscope. Double and triple-positive cells were counted and normalized to UEA-I-positive vascular area using FIJI software (v1.54b, NIH). Further antibody details are listed in Supplementary Table 3 . In vivo cell proliferation assay To evaluate cell proliferation in vivo, we visualized the incorporation of 5-ethynyl-2’-deoxyuridine (EdU), detecting cells undergoing DNA replication. EdU was injected intraperitoneally at 50 mg/kg, 24 h before tissue harvest. EdU incorporation was detected using the click-iT EdU imaging kit (Life Technologies, cat#C10337) according to the manufacturer’s instructions. The number of EdU+ nuclei within the CD31 + vessels were counted and expressed as a percentage of the total number of EC nuclei. Intestinal muscularis whole-mount preparations For intestinal muscularis preparations, the gastrointestinal tract (GIT) was dissected, and the mesenteries were removed. The GIT was straightened and fixed in 10% formalin overnight at 4 °C. Approximately 2 cm of the jejunum was opened longitudinally, and the muscle layer was carefully separated from the underlying submucosa and mucosal tissue under a dissecting microscope using watchmaker forceps. Tissue was stored in PBS at 4 °C until it was processed for whole-mount immunofluorescent staining. Whole-mount immunofluorescence staining and vascular analysis Specimens for whole-mount staining (subcutaneous tissue of postnatal mice and intestinal muscle tissue) were permeabilized and blocked in 5% BSA containing 0.3% Triton X-100 in PBS for 2 h at RT. Tissues were incubated overnight at 4 °C with primary rat anti-mouse CD31 antibody (BD Biosciences, cat#550274, clone MEC 13.3, 0.075 µg/mL). Subsequently, tissues were incubated for 4 h with biotinylated goat anti-rat antibody (Vector laboratories, cat#BA-9401, 7.5 µg/mL) at RT. Biotinylated secondary antibody was detected by incubation with Texas Red® Streptavidin (Vector laboratories, cat#SA-5006-1, 5 µg/mL) for 2 h at RT. For erythrocyte extravasation analysis, tissue was incubated overnight at 4 °C with A647-conjugated anti-mouse TER119 antibody (Biolegend, cat#116218, clone TER-119, 5 µg/mL). For platelet accumulation assessment, tissue was incubated overnight at 4 °C with PE-conjugated CD41 (BD Biosciences, cat#558040, clone MWReg30, 1 µg/mL) or rabbit anti-CD42b (Abcam, cat#183345, clone SP219, 0.3 µg/ml). Subsequently, tissues were incubated for 4 h with goat anti-rabbit A594 antibody (Invitrogen, cat#A32740, 8 µg/mL) at RT. For nuclear counterstaining, tissues were incubated with DAPI (Invitrogen, cat#D1306, 5 µg/mL) for 10 min at RT. Specimens were mounted with Fluoromount-G® mounting medium (Southern Biotech, cat#0100-01). Further antibody details are listed in Supplementary Table 3 . Quantification and visualization of the vasculature in whole-mount preparations For quantification of the vasculature, z-stack images were acquired with Nikon Elements software on a Nikon A1R laser-scanning confocal microscope. A minimum of 3-8 randomly assigned regions were imaged per animal. FIJI (v1.54b, NIH) software was used to reconstruct the Z series as maximum intensity projection. The vascular area was quantified using Angiotool (NIH software) [65] and referred as percentage of the respective total tissue surface area. For vascular tuft analysis, vascular tufts with an area≥200µm 2 were outlined using FIJI software and the number of tufts as well as tuft area was quantified relative to the total vascular area. To assess blood vessel diameter, a grid was placed over each image. Vessel diameter was measured using FIJI software at locations where grid lines intersected a CD31 + /IB4 + vessel. Three-dimensional reconstructions were made using Imaris software (Bitplane, v9.8). Visualization and analysis of mouse brain vasculature For visualization of brain vascular lumina, 70kD A594-conjugated dextran (Invitrogen) was warmed to 37 °C and perfused through the heart of deeply anaesthetized mice. Subsequently, animals were perfused transcardially with ice-cold PBS, then 4% paraformaldehyde (PFA) and each mouse brain was then rapidly extracted. Tissue was cleared using PACT (passive clarity technique) [66] and embedded in RIMS solution for 3D imaging. Specimens were imaged using two-photon microscopy (Nikon A1R MP) and reconstructed using Imaris software (Bitplane). For quantitative analysis, cryosections (50 µM) were labelled using A488-IB4 (1 µg/mL; Invitrogen) at 4 °C overnight and counterstained with DAPI for 5 min at RT. Sections were mounted with Fluoromount-G® mounting medium (Southern Biotech) and Z-stack images were acquired on a Nikon A1R laser scanning confocal microscope. FIJI software was used to reconstruct the Z series as maximum intensity projection. Vascular tufts (area≥ 200µm 2 ) were outlined, and the tuft area was quantified relative to the total vascular area. Retina and hyaloid whole-mount preparation Eyes from P8 mice were enucleated and fixed in 4% PFA on ice. Retina whole-mount preparations were generated [67] , [68] , [69] and labeled with the following: A488-IB4 and DAPI (1 µg/mL; Invitrogen). Hematologic parameters Blood was collected from the inferior vena cava (IVC) of adult mice. The abdominal cavity was opened and approximately 500μL of blood was drawn in a 27-gauge syringe pre-loaded with 50uL of 0.105 M sodium citrate as anticoagulant. Samples were analyzed for blood counts using a Hemavet 950 instrument (Drew Scientific). To obtain plasma, samples were centrifuged at 1100 G for 10 min at RT and plasma was stored at −80 °C. Plasma D-dimer (Asserachrom® D-Di, Diagnostica Stago, cat# NC9884012) levels were determined by enzyme-linked immunosorbent assays following manufacturer’s instructions. Blood smears were prepared via the ‘push’ (wedge) method by placing a small drop (4-6μL) of blood on a slide, spreading the drop using another slide at a 30-45° angle to create a thin smear with a feathered edge, and allowing the smears to air dry for at least 30 min. They were then Wright-Giemsa stained with the Bayer HEMA-TEK2000 slide stainer and imaged at 100x with oil immersion. Between 5-9 photos were taken per mouse with schistocytes and polychromasia quantified per high power field and averaged. Bone marrow analysis Bone marrow (BM) cells were obtained after BM was flushed, treated with red blood cell lysis buffer (150 mM NH 4 CL and 10 mM KHCO 3 ) and washed with staining media (Hank’s Buffered Salt Solution supplemented with 2% fetal bovine serum) [39] . 8 × 10 6 unfractionated BM cells were stained with unconjugated rat lineage-specific antibodies (Ter119, Mac1, Gr-1, B220, CD5, CD3, CD4, CD8) followed by staining with goat anti-rat PE-Cy5 antibody. Cells were then stained using c-Kit-APC-eFluor780, Sca1-PB, CD48-BV711, CD150-PE, Flt3-Biotin, FcgR-PerCP-eFluor710, CD34-FITC, CD41-BV605, and CD105-APC antibodies. Secondary staining was performed with streptavidin-PE-Cy7. Zombie NIR fixable viability kit (BioLegend) was used for dead cell exclusion. Data were collected on a 5 laser Aurora spectral flow cytometer (Cytek Biosciences). Data analysis was performed using FlowJo (BD biosciences) software. Further antibody details are listed in Supplementary Table 5 . 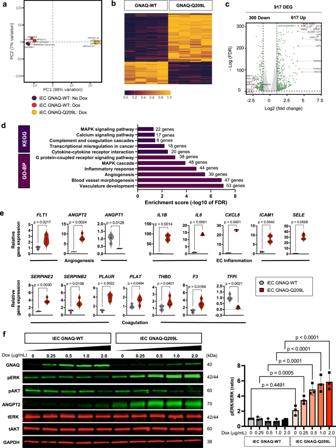Fig. 5: RNA-Sequencing of iECGNAQ-Q209L reveals enriched expression of genes related to angiogenesis, MAPK signaling, inflammatory response, and coagulation. aPrincipal Component Analysis (PCA) of RNA-sequencing data obtained from iECGNAQ-WT no Dox, iECGNAQ-WT + Dox and iECGNAQ-Q209L + Dox.biECGNAQ-WT and toGNAQ-Q209L (n = 4 biological replicates per group) were treated with 1 µg/mL doxycycline for 24 h and total RNA was collected for RNA-seq analysis. Differentially expressed genes (DEG) are defined as log2 (fold change) ≥1 and adjustedPvalue of <0.05. Heat maps of differentially expressed transcripts in iECGNAQ-Q209L compared toGNAQ-WT. Wald test for hypothesis testing.cVolcano-plot of DEGs in iECGNAQ-Q209L compared toGNAQ-WT. A total of 617 genes showed increased expression while 300 genes showed decreased expression in iECGNAQ-Q209L compared to iECGNAQ-WT.dKEGG and GO-BP pathway analyses of DEGs.eA selected group of DEGs were validated using RT-qPCR.n= 4 samples/group(median and quartiles), unpaired two-tailed Welch’s t-test.fRepresentative immunoblots of GNAQ, phospho-ERK (pERK, Thr202/Tyr204), total ERK (tERK), phospho-AKT (pAKT, Ser473), total AKT (tAKT), ANGPT2, and GAPDH in iECGNAQ-WT andGNAQ-Q209L 48 h after doxycycline induction (0, 0.25, 0.5, 1 and 2 μg/ml of Dox). The expression of pERK was quantified and normalized to tERK expression (n= 3 independent experiments). Mean±SD, one-way ANOVA with Tukey’s multiple comparisons. P-values for statistical analysis between all groups are listed in the Source data file. Source data for (c,d,e,f) are provided as a Source Data file. Miles assay For in vivo permeability assay, the dorsal flank of adult mice (6–8 weeks) was bilaterally shaved 24 h prior the experiment. The next day, the histamine H1 receptor antagonist pyrilamine maleate salt (4 mg/kg body weight in 0.9% saline) was injected i.p. 30 min before Evans blue injection to block the effects of local histamine release due to injection-induced mast cell activation. Evans blue (100 µL of 1% in sterile saline) were injected into the tail vein and allowed to circulate for 20 min. VEGF (100 ng/50 µL, R&D Systems) and PBS were injected intradermally into the dorsal flanks. Twenty minutes later, mice were sacrificed by cervical dislocation and the dorsal skin was excised. The weight of the excised skin tissue was noted, and the samples were dried overnight by placing them into 1.5 mL tubes inside a heating block at 55 °C. Evans blue was extracted from the excised tissue by immersion in formamide for 24 h at 55 °C and the amount of blue dye was quantified by spectrometry at 620 nm. The measured OD of each sample was normalized by the weight of the excised tissue and shown as change (ΔOD620) of VEGF-A-treated tissue relative to PBS-treated tissue. Lentiviral vector Full-length wild-type human GNAQ cDNA was purchased from Sino Biologicals (cat# HG17607-U, Wayne, PA) in a pUC19 cloning vector. The specific mutation in c.626 A > T (p.Gln209Leu), was introduced by site-directed mutagenesis using the Q5® Site-Directed Mutagenesis Kit (New England BioLabs Inc., cat#E05545) (Supplementary Fig. 19 ). The following primers were used to introduce the c.626 A > T mutation: Forward 5′-GTAGGGGGCCtAAGGTCAGAG −3′, and Reverse 5′- ATCGACCATTCTGAAAATGACAC −3′. The GNAQ WT and Q209L cDNA was subsequently introduced into the lentiviral vector pCW-Cas9 (pCW-Cas9 was a gift from Eric Lander & David Sabatini (Addgene plasmid # 50661; http://n2t.net/addgene:50661 ; RRID:Addgene_50661), at NheI(5’) and BamHI I (3’) to replace the Cas9 gene. The lentivirus was generated by using second-generation packaging system at the Cincinnati Children’s Hospital viral vector core facility. Lentiviral transduction of human endothelial cells Human endothelial colony-forming cells (ECFC, StemBiosys) were plated onto fibronectin-coated (1 µg/cm 2 , Sigma, cat#FC010) plates and cultured in endothelial growth medium (EGM2, Lonza, cat# CC-3162) supplemented with 10% fetal bovine serum (FBS) (GE Healthcare, cat#SH30910.03) and 1% penicillin-streptomycin-glutamine (Corning, Cat#30-009-CI). Cells were treated with Hexadimethrine bromide (8 μg/mL, Sigma, cat# TR-1003-G) and lentiviral particles containing pCW- GNAQ -WT or pCW- GNAQ -Q209L were added. After 24 h the media was replaced with puromycin (1 μg/mL, Gibco, cat#A1113803) containing media to select for cells that had taken up the constructs. Lentiviral-engineered ECFC expressing WT or Q209L GNAQ cDNA were designated as iEC GNAQ -WT and iEC GNAQ -Q209L, respectively. Doxycycline (Dox, Sigma, cat#D3447) was added to the media to induce GNAQ -WT or GNA Q-Q209L expression (0.25-2 μg/mL) for 48 h before cells were lysed for Western Blot analysis. For inhibitor studies, cells were treated with 1 nM, 5 nM or 10 nM Trametinib or vehicle (DMSO 1 µL/mL) for 20 min. Immunofluorescence monolayer staining for VE-cadherin Immunofluorescence staining was performed on 4% PFA fixed ECFC monolayers with an A647-conjugated VE-Cadherin antibody (BD Biosciences, cat#561567, 0.5 µg/mL), for 2 h at RT. For nuclear counterstaining, cells were incubated with DAPI (Invitrogen, D1306, 5 µg/mL) for 10 min at RT. Specimens were mounted with Fluoromount-G® mounting medium (Southern Biotech, cat#0100-01). Z-stack (10 µM) confocal images were acquired on a Nikon A1R laser scanning confocal microscope. For quantification, VE-Cadherin positive area was measured using FIJI software (v1.54b, NIH) and normalized to the number of cells. Cells from n = 5 independent experiments (for each experiment n = 10 images) were used for quantifications. Immunoblotting Cells were washed with PBS then lysed using ice-cold RIPA lysis buffer (Boston Bioproduct) supplemented with HALT TM protease/phosphatase inhibitor cocktail (Thermo Scientific, cat# 78442). The protein concentration was determined using the BCA Protein Assay Kit (Thermo Scientific, cat# PI23225). 20 µg of total protein were subjected to SDS-PAGE (4-20%, Midi Criterion precast gels, Bio-Rad, cat#5678094) and transferred to a PVDF membrane (Immobilon®-P PVDF Membrane, Millipore, cat#IPVH00010). Membranes were blocked for in 5% nonfat dried milk for 1 h at RT and probed with the following antibodies: rabbit anti-GNAQ (Cell Signaling, cat#14373, clone D5V1B 0.05 µg/mL), mouse anti-VE-Cadherin (Santa Cruz, cat# sc-9989, clone F-8, 0.5 µg/mL), rabbit anti-pERK 1/2 (Thr202/Tyr204, Cell Signaling, cat#9101, polyclonal, 0.5 µg/mL), mouse anti-ERK 1/2 (Cell Signaling, cat#4696, clone L34F12, 0.5 µg/mL), rabbit anti-pAKT (Ser473, Cell Signaling, cat#4060, clone D9E, 0.5 µg/mL) and mouse anti-AKT (Cell signaling, cat#2920, clone 40D4, 0.2 µg/mL), goat anti-Angiopoietin-2 (R&D Systems, cat#AF-623, polyclonal, 1 µg/mL) and mouse anti-GAPDH (Millipore, cat# MAB374, clone 6C5, 0.2 µg/mL). Membranes were incubated with the following secondary antibodies: Donkey anti-mouse IgG-DyLight TM 680 (Invitrogen, cat# SA5-10170, 0.1 µg/mL), goat anti-rabbit IgG-DyLight TM 800 (Invitrogen, cat#SA5-10036, 0.1 µg/mL) or donkey anti-goat IgG-DyLight TM 800 (Invitrogen, cat#SA5-10092, 0.1 µg/mL). Antigen–antibody complexes were visualized using Odyssey Scanner and analyzed using Image Studio Software (LI-COR, v5.2). Further antibody details are listed in Supplementary Table 3 . RNA isolation and RNA sequencing Cells were cultured in 2% FBS EGM2 containing 1 µg/mL doxycycline for 18 h. Cells were treated with Trametinib (10 nM, LC laboratories, cat#T-8123) or vehicle for additional 6 h. Total RNA was extracted using RNeasy extraction kit (Qiagen) according to manufacturer’s recommendations. RNA integrity number and concentration was assessed using a 5300 Fragment Analyzer System (Agilent) at the DNA Sequencing and Genotyping Core. 300 ng of total RNA was used for library preparation using the Illumina Stranded mRNA Prep—Ligation kit. 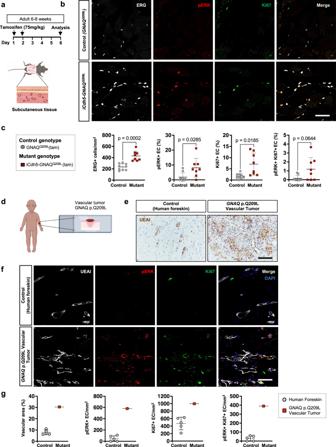Fig. 6: Increased ERK activation in the vasculature ofGNAQQ209Lexpressing mice and patient vascular tumor. aTamoxifen induction scheme for analysis of subcutaneous tissue.bRepresentative images of subcutaneous tissue of tamoxifen-treated control andiCdh5-GNAQQ209Lmutant mice stained for ERG (white), pERK (red), Ki67 (green), and merge. Scale bar: 50 μm.cERG staining marks EC nuclei. Quantification of ERG+cells normalized per subcutaneous tissue area. pERK+and Ki67+and double-positive endothelial cells were normalized to total EC number.iCdh5-GNAQQ209L(n= 9) and control littermates (n= 9), mean±SD, unpaired two-tailed Welch’s t-test. Mouse genotypes are indicated.dGNAQQ209Lmutant patient-derived vascular tumor tissue was analyzed.eRepresentative images of neonatal human foreskin and patient-derived tissue (cutaneous vascular tumor) with somaticGNAQp.Q209L mutation immuo-stained for UEAI (Ulex europaeus agglutinin-I) (brown). Scale bar: 50μm.fRepresentative images of neonatal human foreskin and patient-derived tissue with somaticGNAQp.Q209L mutation labeled for UEAI (white), pERK (red), Ki67 (green), and merge with DAPI (blue). Scale bar: 50 μm.gQuantification of the UEAI+vascular area as percentage of total field area, pERK+, Ki67+and double-positive EC calculated as events per mm2of vascular area; human foreskin tissue fromn= 5 different donors, andn= 1 patient-derived tumor tissue, mean±SD. Source data for (c,g) are provided as a Source Data file. Schematic in (a,d) created with Biorender.com. 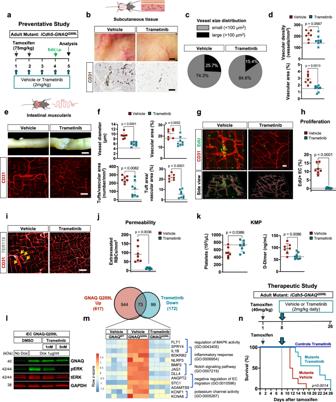Fig. 7: Trametinib treatment ofGNAQQ209Lmutant mice rescues vascular phenotype, hyperproliferation, permeability and coagulopathy. aPreventative study scheme. 6 weeks-oldiCdh5-GNAQQ209Lmice induced with 75 mg/kg tamoxifen and concomitantly treated with Trametinib (2 mg/kg/day) or vehicle.bMacroscopic photographs of subcutaneous tissue from vehicle and Trametinib -treated mice. CD31 (dark brown) stained tissue sections. Scale bars: 2 mm and 50μm.cVessel size distribution in subcutaneous tissue as percentage of small (<100 µm2) and large (>100 µm2) vessels.dVascular density and area in vehicle or Trametinib -treated mice.eRepresentative photograph of intestine from vehicle and Trametinib -treatediCdh5-GNAQQ209Lmice. Whole-mount intestinalmuscularisstained for CD31 (red), z-stack maximum intensity projection. Scale bars: 2 mm and 100 μm.fQuantification of intestinalmuscularisvessel diameter, vascular area, tuft number and tuft area.gIntestinal whole-mounts labeled for EdU (green) and CD31 (red). Scale bar: 20μm.hEdU positive EC (EdU+/CD31+) as percentage over total EC number (CD31+).iRepresentative z-stack maximum intensity projection of intestinalmuscularisstained for TER119 (white) and CD31 (red). Yellow arrows indicate extravasated erythrocytes. Scale bar: 100μm.jQuantification of extravasated erythrocytes normalized to tissue area.kPlatelet counts and D-Dimer levels in vehicle or Trametinib -treatediCdh5-GNAQQ209Lmice. Ind,f,h,jandk: vehicle (n= 7), Trametinib(n= 8), mean±SD, unpaired two-tailed Welch’s t-test. Black dotted lines indicate reference values in untreated control mice.lRepresentative immunoblot of iECGNAQ-Q209L treated with DMSO or Trametinib and probed for GNAQ, phosphor-ERK (pERK, Thr202/Tyr204), total ERK (tERK), and GAPDH (n= 3 independent experiments).mVenn diagram of genes upregulated in iECGNAQ-Q209L and downregulated with Trametinib treatment (6 h). Expression levels of 73 genes were normalized by Trametinib (adjustedP-value of <0.05 and a log2 (fold change) >1). Heatmap of selected genes clustered by GO-terms. Wald test for hypothesis testing.nTherapeutic study scheme. 6 weeks-oldiCdh5-GNAQQ209Lmice induced with 40 mg/kg tamoxifen and after 8 days treated daily with Trametinib (2 mg/kg) or vehicle. Kaplan-Meier survival curve of vehicle (n= 8, red) and Trametinib -treated (n= 9, turquoise)iCdh5-GNAQQ209Lmice. Gehan-Breslow-Wilcoxon test. Trametinib-treated control mice (iCdh5mice,n= 3, blue). Source data for (c,d,f,h,j,k,l,m,n) are provided as a Source Data file. Schematic in (b,e) created with Biorender.com. The libraries were then quantified and sequenced using an Illumina NovaSeq 6000 at a sequencing depth of 40 million reads per sample. RNA-seq reads in FASTQ format were first subjected to quality control to assess the need for trimming of adapter sequences or bad quality segments. The programs used in these steps were FastQC v0.11.7 ( http://www.bioinformatics.babraham.ac.uk/projects/fastqc ), Trim Galore! v0.4.2 ( https://www.bioinformatics.babraham.ac.uk/projects/trim_galore ) and Cutadapt v1.9.1 [70] . The trimmed reads were aligned to the reference human genome version hg38 with the program STAR v2.6.1e [71] . Aligned reads were stripped of duplicate reads with the program Sambamba v0.6.8 [72] . Gene-level expression was assessed by counting features for each gene, as defined in the NCBI’s RefSeq database [73] . Read counting was done with the program featureCounts v1.6.2 from the Rsubread package [74] . Raw counts were normalized as transcripts per million (TPM). Differential gene expressions between groups of samples were assessed with the R package DESeq2 v1.26.0 [75] . Gene list and log2 fold change are used for GSEA analysis using GO pathway dataset [76] , [77] . Plots were generated using the ggplot2 v3.3.6 [78] package and base graphics in R. Heatmaps were created using pheatmap (RRID:SCR_016418, v1.0.12.). Gene ontology (GO) and Kyoto Encyclopedia of Genes and Genomes (KEGG) pathway analyses were performed using ShinyGO (V.0.76.2) [79] where adjusted p value (FDR) cut-off was set on 0.05. RNA-seq data was submitted to the Gene Expression Omnibus (GEO) (Accession number: GSE216367 ). Real-time reverse transcriptase PCR Reverse transcriptase reactions were performed using an iScript cDNA synthesis kit (Bio-Rad, cat#1708841). qPCR was performed using SsoAdvanced Universal SYBR(R) Green Supermix (Bio-Rad, cat#1725272). Amplification was performed in Bio-Rad Touch Real-time PCR detection system (CFX96). 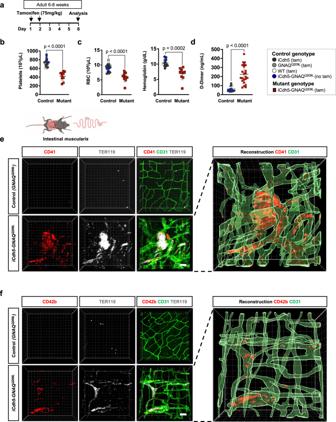A relative standard curve of each gene amplification was generated and an amplification efficiency of >90% was considered acceptable. Hypoxanthine phosphoribosyl transferase 1 ( HPRT1 ) and TATA-binding protein 1 ( TBP1 ) were used as housekeeping genes. Quantification was performed using the Pfaffl method [80] . Fig. 4: Mice expressingGNAQQ209Lin the vasculature develop thrombocytopenia and severe coagulopathy. aTamoxifen induction scheme.b-cHematological parameters were measured iniCdh5-GNAQQ209L(n= 10) and controls (n= 18), mean±SD, unpaired two-tailed Welch’s t-test. Mouse genotypes are indicated.bPlatelet counts,cRBC (red blood cell counts), and hemoglobin levels.dD-Dimer levels were measured in plasma samples fromiCdh5-GNAQQ209L(n= 23) and controls (n= 28), mean±SD, unpaired two-tailed Welch’s t-test. Mouse genotypes are indicated.e-fRepresentative confocal z-stack images (max. intensity projection) of intestinalmuscularisstained foreCD41 orfCD42b (red) together with CD31 (green) and TER119 (white/grey). Images are representative ofn= 3 mice/group and were 3D reconstructed. Scale bar: 40μm. Source data for (b,c,d) are provided as a Source Data file. Schematic in (e) created with Biorender.com. Primer sequences are shown in Supplementary Table 4 . Data collection and statistics Excel (v16.67) was used to collect and organize raw data. Prism 9.0 software (GraphPad Software, v9.3.1) was used for all statistical assessments. Data analyzed statistically are presented as mean±standard deviation (SD) of two or more biological replicates ( n values reported in figure legends). Statistical significance between two groups was assessed by parametric Welch’s t-test. When more than two groups were compared, one or two-way ANOVA was used followed by Tukey, Dunnett’s or Sidak’s post hoc test. Differences were considered significant for P value less than 0.05. Schematics in all figures were created using Biorender.com. Reporting summary Further information on research design is available in the Nature Portfolio Reporting Summary linked to this article.